Global 3′ UTR shortening has a limited effect on protein abundance in proliferating T cells Alternative polyadenylation is a cellular mechanism that generates mRNA isoforms differing in their 3′ untranslated regions (3′ UTRs). Changes in polyadenylation site usage have been described upon induction of proliferation in resting cells, but the underlying mechanism and functional significance of this phenomenon remain largely unknown. To understand the functional consequences of shortened 3′ UTR isoforms in a physiological setting, we used 3′ end sequencing and quantitative mass spectrometry to determine polyadenylation site usage, mRNA and protein levels in murine and human naive and activated T cells. Although 3′ UTR shortening in proliferating cells is conserved between human and mouse, orthologous genes do not exhibit similar expression of alternative 3′ UTR isoforms. We generally find that 3′ UTR shortening is not accompanied by a corresponding change in mRNA and protein levels. This suggests that although 3′ UTR shortening may lead to changes in the RNA-binding protein interactome, it has limited effects on protein output. Expression of messenger RNA (mRNA) precursors transcribed by RNA polymerase II requires recognition and processing of signals in the pre-mRNA by the cleavage and polyadenylation factors to guide proper formation of 3′ ends. Most mammalian genes have multiple polyadenylation (poly(A)) sites [1] , [2] , whose regulated selection leads to the production of alternative mRNA forms that differ in localization, stability and/or protein-coding potential. A systematic shift towards coding region-proximal 3′ end processing sites, leading to an overall shortening of 3′ untranslated regions (3′ UTRs) was recently observed in activated compared with naive lymphocytes [3] as well as in cells that proliferate rapidly [4] , [5] . The differentiation of embryonic stem cells and, conversely, the induction of pluripotency in somatic cells, are associated with changes in opposite directions in 3′ UTR lengths [2] , [6] , [7] . The functional significance of this regulation is not well understood. Initial studies suggested that the lack of microRNA (miRNA)-binding sites in the shortened 3′UTRs leads to an increased stability of the mRNAs and an increased protein output [3] , [4] . This conjecture was later refuted by a transcriptome-wide analysis that was carried out in mouse embryonic fibroblasts, where small differences in the relative stability of 3′ UTR isoforms were found [8] . MiRNAs are only one class of regulators that act on 3′ UTRs, guiding the RNA-induced silencing complexes to target mRNAs to increase their decay rate and reduce translation [9] , [10] . The 3′ UTRs contain binding sites for many RNA-binding proteins (RBPs) and integrate a variety of signals for mRNA localization, decay and translation. Of the hundreds of RBPs that bind and potentially regulate various aspects of mRNA metabolism [11] , [12] , at least some, such as the human antigen R (HuR) [13] and the A/U-rich-element-binding factor-1 (also known as the heterogeneous nuclear ribonucleoprotein D or hnRNPD) [14] , have been reported to increase mRNA stability. A very recent study that was carried out in yeast [15] found that the stability of transcripts is not correlated with the length of their 3′ UTRs. However, the protein that appeared to cause the largest difference in decay rates between 3′ UTR isoforms in this study, Puf3, had an overall destabilizing effect (presumably on the longer 3′UTR isoforms, containing additional Puf3-binding sites compared with the shorter 3′ UTR isoforms). Thus, the functional relevance of the observed systematic reduction in 3′ UTR lengths in relation to cell proliferation remains unclear. To determine the consequences and functional relevance of 3′ UTR shortening during lymphocyte activation, we undertook a systematic investigation of the changes in the poly(A) site usage and in the protein output of the corresponding genes in mouse and human T cells. Activated T cells express mRNAs with shortened 3′ UTRs We focused our investigation on the T cell activation system, in which the 3′ UTR shortening was initially described [3] . We dissected spleen and lymph nodes from C57BL/6 mice and isolated T cells by MACS purification. T cells were activated for 72 h with CD3/CD28 Dynabeads and IL-2 (see Methods) and libraries of 3′ ends of mature mRNAs were prepared and processed with the A-seq protocol as described previously [16] . 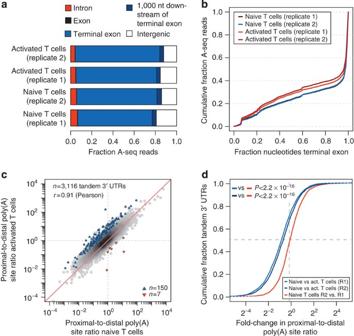Figure 1: 3′ end sequencing reveals increased proximal poly(A) site usage upon activation of murine T cells. (a) Annotation of reads obtained from mRNA 3′ end sequencing of naive and activated T cells. Two biological replicates were used for each condition. (b) Coverage of terminal exons by 3′ end sequencing reads as a function of the distance from the exon start. Activated T cells show increased coverage of the 5′ compared with the 3′ region of terminal exons, resulting from preferential use of proximal poly(A) sites. (c) Contour plot of the relative use of proximal and distal poly(A) sites in naive and activated T cells. Only genes with tandem poly(A) sites are shown. Genes that were identified to undergo significant changes in poly(A) site use are marked by coloured triangles with blue indicating increased use of the proximal poly(A) site and red indicating increased use of the distal poly(A) site in activated T cells. (d) Cumulative distribution function of the change in proximal vs distal poly(A) sites between pairs of samples (data shown inc). The shift towards increased usage of proximal poly(A) sites is statistically highly significant (P-values obtained by Mann–Whitney test on 3,116 genes with tandem poly(A) sites). Excluding reads that may result from internal priming, we identified 269,751 high-confidence poly(A) sites in the mouse genome, to which a total of 32,388,835 reads mapped ( Supplementary Table 1 ). For each library, more than 70% of the reads mapped to terminal exons of transcripts and only a small fraction (less than 0.5%) to other exons ( Fig. 1a ). Compared with resting T cells, the density of 3′ end sequencing reads in terminal exons showed a clear and highly reproducible shift towards the 5′ end of terminal exons in the activated T cells ( Fig. 1b ). Figure 1: 3′ end sequencing reveals increased proximal poly(A) site usage upon activation of murine T cells. ( a ) Annotation of reads obtained from mRNA 3′ end sequencing of naive and activated T cells. Two biological replicates were used for each condition. ( b ) Coverage of terminal exons by 3′ end sequencing reads as a function of the distance from the exon start. Activated T cells show increased coverage of the 5′ compared with the 3′ region of terminal exons, resulting from preferential use of proximal poly(A) sites. ( c ) Contour plot of the relative use of proximal and distal poly(A) sites in naive and activated T cells. Only genes with tandem poly(A) sites are shown. Genes that were identified to undergo significant changes in poly(A) site use are marked by coloured triangles with blue indicating increased use of the proximal poly(A) site and red indicating increased use of the distal poly(A) site in activated T cells. ( d ) Cumulative distribution function of the change in proximal vs distal poly(A) sites between pairs of samples (data shown in c ). The shift towards increased usage of proximal poly(A) sites is statistically highly significant ( P -values obtained by Mann–Whitney test on 3,116 genes with tandem poly(A) sites). Full size image To further validate the quality and reproducibility of our results, we compared libraries on gene-by-gene basis using the number of reads mapped to terminal exons of transcripts assigned to a particular gene as a proxy for the expression level of a gene. Requiring a minimal expression level of five reads per million in at least one of the four libraries, we identified 9,928 genes as being expressed in naive and activated murine T cells. Biological replicates of both naive and activated T cells showed very high correlation ( r ≥0.94; Supplementary Fig. 1 ). 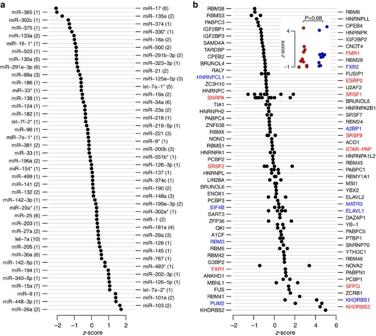Figure 2: Quantification of the loss of regulatory elements upon 3′ UTR shortening. Influence of 3′ UTR shortening on miRNA (a) and RBP (b) target sites. Thexaxis represents thez-score of the loss of binding sites obtained by comparing the observed loss of target sites with what would be expected from random permutations of target sites across the set of alternative 3′ UTRs. A negativez-score indicates that the loss in binding sites is greater than if sites were placed randomly in alternative regions of 3′ UTRs. RBPs with a stabilizing effect on their transcript targets as assigned in Rayet al.32are marked in blue, whereas RBPs with a destabilizing effect are marked in red. The inset showsz-scores obtained for representative PWMs of RBPs with stabilizing and destabilizing effects (P-value obtained from a Wilcoxon rank sum test). The genes that were upregulated in activated T cells showed a clear enrichment of cell cycle-associated Gene Ontology (GO) terms, whereas immune system-related GO terms were most enriched among downregulated genes ( Supplementary Table 2 ). These results are consistent with the physiological state of the cells and further demonstrate that our 3′ end sequencing data accurately reflect transcript-level changes. To investigate the dynamics of 3′ end processing, we first clustered the poly(A) sites that were very closely spaced and probably the result of imprecise 3′ end cleavage and identified distinct poly(A) sites [16] . The nucleotide distribution in regions flanking the inferred sites and the presence of upstream polyadenylation signals indicate that our strategy allowed us to identify genuine poly(A) sites ( Supplementary Fig. 2A,B ). We then restricted our analysis to tandem poly(A) sites that were located in the same terminal exon, as was done in a previous study [3] . 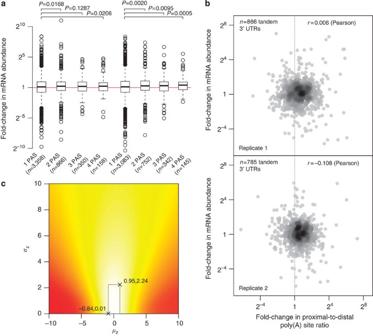Figure 3: Evaluation of changes in mRNA levels in naive and activated murine T cells with respect to changes in poly(A) site usage. (a) Comparison of fold-changes in mRNA abundance for genes with a single or multiple poly(A) sites (PAS;P-values obtained from a one-sidedt-test). (b) Correlation between changes in mRNA abundance and changes in poly(A) site usage. The centre of mass of the cloud of points is at a positivex-value, reflecting the noted increase in proximal poly(A) site use in dividing cells. (c) Contour plot of the log-likelihood of the data as a function of the mean and standard deviation of the log ratio of decay rates (z) of the short and long 3′ UTR isoforms. The colour gradient ranging from red to white describes the log likelihood obtained under the model, with white values showing the better fit. The box marks the 95% posterior probability interval of the parameters (μz,σz). Overall, we inferred that 3,116 genes undergo alternative polyadenylation (APA) at tandem poly(A) sites ( Supplementary Table 3 ). The number of reads assigned to poly(A) sites in the 5′ half and the 3′ half of terminal exons showed good reproducibility between biological replicates indicating that our data can be used to analyse the relative use of alternative poly(A) sites in different conditions ( Supplementary Fig. 2C ). As expected from a previous study [3] , there was a marked shift towards increased usage of proximal poly(A) sites in activated compared with naive T cells ( Fig. 1c ). The shift is not restricted to a small subset of genes, but affected the entire transcriptome ( Fig. 1d ). That is, more than 70% of genes showed an increased use of proximal poly(A) sites upon T cell activation. We used the DEXSeq software to analyse the differential use of poly(A) sites [17] . 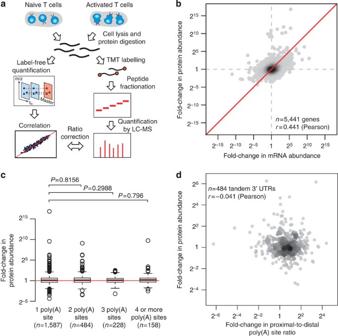Figure 4: Influence of 3′ UTR shortening on protein levels in murine T cells. (a) Quantitative mass spectrometry (liquid chromatography-mass spectrometry (LC-MS))-based proteomics workflow. Proteins extracted from naive and activated mouse and human T cells were digested and subjected to label-free and tandem mass tag (TMT) quantification, respectively. The TMT-labelled peptides were further fractionated using isoelectric focusing before LC-MS analysis to increase proteome coverage. Finally, the ratios obtained by the TMT approach were correlated with the label-free quantities to correct for possible ratio distortion effects in the final TMT-based quantitative data sets, which comprised more proteins than the data sets based on LFQ. (b) Correlation of mRNA and protein abundance changes between activated and naive T cells. (c) Change in protein abundance between activated and naive T cells for genes with one to four or more tandem poly(A) sites. (d) Correlation between the change in proximal poly(A) site use and the change in protein level. A total of 157 genes showed a significant difference ( P -value ≤0.05) in the proximal-to-distal poly(A) site use between naive and activated T cells ( Supplementary Table 4 ), and 150 of these genes (96%) had an increased abundance of proximal transcript isoforms in activated T cells. This set includes Bcl2 , Creb1 and Tnfrsf9 (CD137), genes that are known to influence proliferation [18] , [19] , [20] . Whereas the increased proximal poly(A) site use of Bcl2 and Tnfrsf9 is associated with increased expression, consistent with the initial reports of the effect of 3′ UTR shortening on gene expression, the expression of Creb1 , is rather reduced, at least at the mRNA level. An example of a gene with a marked shift towards increased proximal poly(A) site use upon T cell activation is shown in Supplementary Fig. 3A , which depicts a CLIPZ [21] genome browser screenshot of the 3′ UTR of Reep5 . It is well known that upon activation, T cells undergo a dramatic remodelling of the cytoskeleton [22] . Some of the genes that are involved in this process also show a significantly higher use of proximal poly(A) sites. These are Pak1 and Prkca (PKCα), which are involved in signalling transduction cascades, as well as Wasf2 (WAVE2) [23] , Marcks [24] or Jmy [25] , which interact directly with actin. Again in contrast to the expectation that the stability of short 3′ UTR isoforms is higher compared with the long 3′ UTR isoforms [4] , all of these immune response-related genes are downregulated at the mRNA level, in spite of their increased use of proximal poly(A) sites. Moreover, when we analysed separately genes that are significantly downregulated or upregulated at the mRNA level upon T cell activation, we found that downregulated genes showed a more pronounced 3′ UTR shortening than upregulated genes ( Supplementary Fig. 3B ). This motivated us to investigate the relation between the change in poly(A) site use and the change in mRNA/protein abundance in more detail. Regulatory element content of 3′ UTR isoforms Among the regulatory elements that are lost when proximal poly(A) sites are used more frequently, are binding sites for miRNAs that in naive T cells could contribute to the repression of gene expression [3] . 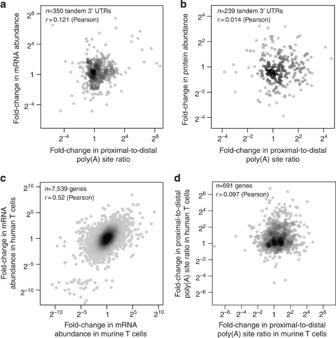Figure 5: Evolutionary conservation of alternative polyadenylation at tandem poly(A) sites. Assessment of the impact of 3′ UTR shortening on mRNA (a) and protein (b) levels in naive and activated human T cells. (c) Comparison of changes in mRNA levels upon T cell activation in murine and human T cells. (d) Comparison of changes in poly(A) site use upon T cell activation in murine and human T cells. Only orthologous genes that showed the same number of alternative poly(A) sites in mouse and human were considered. To assess the consequence of 3′ UTR shortening on the miRNA-mRNA interactome of T cells, we retrieved miRNA target predictions from the ElMMo database [26] and counted the number of target sites for each miRNA seed family in the common and alternative parts of the 3′ UTRs of genes with tandem poly(A) sites ( Supplementary Table 5 ). MiRNA target sites that are located between the most proximal and most distal poly(A) site in the alternative 3′ UTR region constitute a significant fraction of all predicted target sites. This is a reflection of the large change in 3′ UTR length that is associated with T cell activation. For example, 65% of all the target sites predicted for the miR-29a seed family are located in the alternatively processed region of the 3′ UTRs. To examine which miRNA regulators would be most affected by 3′ UTR shortening, we carried out the following test. Each site predicted by ElMMo has an associated probability of being under evolutionary selection. By summing the probabilities of individual binding sites in a 3′ UTR, we obtained an expected number of sites that are under selection. Performing this computation for individual transcript isoforms with their corresponding expression levels estimated based on 3′ end sequencing, we obtained expected numbers of sites in the isoforms produced in a specific condition (activated and naive T cells). As expected from a global shortening of 3′ UTRs, we find a net loss of target sites for all miRNAs. However, the loss of target sites by 3′ UTR shortening does not affect all miRNAs to a similar degree. To identify which miRNAs would be most affected by the 3′ UTR shortening, we randomized the predicted interactions involving the alternative parts of 3′ UTRs. This amounts to randomizing the ‘labels’ that indicate which miRNA binds an individual site. Computing the z -score of the observed change in the number of sites relative to what would be expected from the randomized data set, we found large differences between miRNAs. In particular, miRNAs that have been implicated in the regulation of cell proliferation appear at the extreme of the z -score range, some (miR-17, miR-365 and miR-135a [27] , [28] , [29] ) losing more sites than expected and others (miR-26a, miR-103 (refs 30 , 31 ) losing less sites than expected ( Fig. 2a ). MiRNAs with a cell type-specific expression show a less extreme pattern of site loss. These results indicate that APA at proximal poly(A) sites in proliferating cells does impact the susceptibility of the corresponding genes to regulation by miRNAs that themselves are involved in cell proliferation. Figure 2: Quantification of the loss of regulatory elements upon 3′ UTR shortening. Influence of 3′ UTR shortening on miRNA ( a ) and RBP ( b ) target sites. The x axis represents the z -score of the loss of binding sites obtained by comparing the observed loss of target sites with what would be expected from random permutations of target sites across the set of alternative 3′ UTRs. A negative z -score indicates that the loss in binding sites is greater than if sites were placed randomly in alternative regions of 3′ UTRs. RBPs with a stabilizing effect on their transcript targets as assigned in Ray et al . [32] are marked in blue, whereas RBPs with a destabilizing effect are marked in red. The inset shows z -scores obtained for representative PWMs of RBPs with stabilizing and destabilizing effects ( P -value obtained from a Wilcoxon rank sum test). Full size image We similarly evaluated the change in the susceptibility of transcripts to regulation by RBPs. Binding motifs for a relatively large set of RBPs were recently published in the form of positional weight matrices (PWMs) [32] . Based on these PWMs and on the alignments of a number of genomes (see Methods), we predicted evolutionarily conserved RBP-binding sites in the 3′ UTRs of expressed genes with a method that was introduced previously [33] . Applying the procedure that we described above for miRNAs starting from the inferred probabilities of RBP-binding sites to be under evolutionary selection, we determined which RBPs lose the most or least sites upon increased use of proximal poly(A) sites, compared with what we would expect by chance ( Fig. 2b ). As for miRNAs our analysis revealed large differences between individual RBPs. The expected impact of this regulation is, however, more complex because in contrast to miRNAs, for which the evidence for target destabilization is overwhelming [10] , RBPs have a variety of functions. An individual RBP frequently acts at multiple levels of gene regulation, including APA [34] . Nonetheless, Ray et al . [32] have already associated a few of the RBPs from their study with changes in mRNA stability. These proteins are indicated by the red (destabilizers) and blue (stabilizers) colours in Fig. 2b . We do not observe a clear trend of destabilizing RBPs losing more sites and stabilizing RBPs losing less sites than expected by chance, which would be consistent with the small bias of shorter 3′ UTR isoforms being more stable than the corresponding long 3′ UTR isoforms [8] . Two proteins with the best established function in mRNA stabilization, ELAVL1 (HuR) and PUM2 (Pumillio 2), appear to be losing less sites than expected. To facilitate further investigations into the impact of 3′ UTR shortening on the fate of individual mRNAs, we have summarized the transcripts that are predicted to be regulated by those regulators whose impact on the transcriptome is most affected by the systematic change in poly(A) site use ( Supplementary Data 1 ). The impact of 3′ UTR shortening on mRNA abundance The above analysis suggests that, consistent with the conclusions drawn from the initial studies of 3′ UTR shortening [3] , [4] , preferential processing at proximal poly(A) sites in proliferating cells leads to an overall loss of destabilizing sequence elements. This would be expected to lead to increased expression of genes with tandem poly(A) sites, yet it is not what we observed in our initial analysis of genome-wide gene expression changes. We next focused on genes with a simple pattern of polyadenylation, considering only genes with tandem poly(A) sites and genes with a single poly(A) site, and excluding genes with more complex patterns of APA (such as alternative terminal exons). We further restricted our set to genes for which spurious A-seq reads in the rest of the gene body including cryptic intronic sites accounted for at most 10% of the reads that were assigned to main poly(A) sites. We estimated the overall mRNA expression level of each gene as the sum of A-seq reads assigned to poly(A) sites located in the terminal exon. Comparing the change in total mRNA levels between naive and activated T cells for genes with two, three or four tandem poly(A) sites relative to genes with a single poly(A) site, we found a slight trend of upregulation of genes with multiple poly(A) sites in activated cells ( Fig. 3a ). Considering genes with precisely two poly(A) sites, we asked whether the change in total mRNA level can be attributed to the change in the relative use of proximal and distal poly(A) sites. If gene expression was mainly regulated through APA with the short 3′ UTR isoform being significantly more stable than the long isoform, we would expect a positive correlation between the change in the total mRNA level and the change in proximal vs distal polyadenylation site use. As shown in Fig. 3b we did not detect such a relationship. Figure 3: Evaluation of changes in mRNA levels in naive and activated murine T cells with respect to changes in poly(A) site usage. ( a ) Comparison of fold-changes in mRNA abundance for genes with a single or multiple poly(A) sites (PAS; P -values obtained from a one-sided t -test). ( b ) Correlation between changes in mRNA abundance and changes in poly(A) site usage. The centre of mass of the cloud of points is at a positive x -value, reflecting the noted increase in proximal poly(A) site use in dividing cells. ( c ) Contour plot of the log-likelihood of the data as a function of the mean and standard deviation of the log ratio of decay rates ( z ) of the short and long 3′ UTR isoforms. The colour gradient ranging from red to white describes the log likelihood obtained under the model, with white values showing the better fit. The box marks the 95% posterior probability interval of the parameters ( μ z , σ z ). Full size image The observed abundance of short and long 3′ UTR isoforms in different conditions depends not only on the relative rates of polyadenylation at the two sites, but also on the overall rates of transcription and the relative rates of decay of the two transcript forms in the two conditions. To estimate the relative decay rates of short and long isoforms from the 3′ end sequencing data, eliminating the effect of confounding factors, we developed a mathematical model (described in Methods) based on the assumption that the distribution of changes in the transcription rate of genes between activated and naive T cells is similar for genes with a single poly(A) site and genes with two tandem poly(A) sites. The contour plot of the log likelihood of the data for the 712 genes with two tandem poly(A) sites under the model, as a function of the mean and standard deviation of the log-ratio of the decay rates of long and short isoforms is shown in Fig. 3c . We infer that μ z , the average of the log-ratio of decay rates is located between −0.84 and 0.95. Thus, consistent with a recent study in which the decay rates of long and short isoforms were estimated in mouse fibroblasts [8] , we found little evidence for short 3′ UTR isoforms being generally more stable compared with long 3′ UTR isoforms. Because 3′ UTR-mediated interactions with RBPs may also affect the translation rates of mRNAs, we next evaluated the protein output of genes with tandem poly(A) sites in naive and activated T cells. The impact of 3′ UTR shortening on protein abundance To quantify dynamic protein changes on a system-wide level, we combined high mass accuracy mass spectrometry with isobaric tandem mass tagging (TMT) [35] and extensive off-gel electrophoresis sample fractionation ( Fig. 4a ) [36] . Performing our experiment in biological duplicates we obtained a total of 138,816 peptide-spectral matches, 48,113 unique peptides and overall quantified 6,187 protein clusters/genes at 1% false discovery rate. It has been reported that ratio compression arising from co-isolated peptides is prevalent with TMT-labelled peptides and needs to be controlled to achieve accurate protein quantification [37] . Therefore, we carried out additional unbiased, label-free quantifications (LFQs) of all samples. As reported previously [38] , [39] , we observed a good linear correlation of TMT and LFQ protein ratios ( Supplementary Fig. 5A,B ). This suggested that the ratio compression of TMT can be largely corrected by an average compression factor [38] and we therefore recalculated all TMT ratios accordingly (see Supplementary Methods ). Figure 4: Influence of 3′ UTR shortening on protein levels in murine T cells. ( a ) Quantitative mass spectrometry (liquid chromatography-mass spectrometry (LC-MS))-based proteomics workflow. Proteins extracted from naive and activated mouse and human T cells were digested and subjected to label-free and tandem mass tag (TMT) quantification, respectively. The TMT-labelled peptides were further fractionated using isoelectric focusing before LC-MS analysis to increase proteome coverage. Finally, the ratios obtained by the TMT approach were correlated with the label-free quantities to correct for possible ratio distortion effects in the final TMT-based quantitative data sets, which comprised more proteins than the data sets based on LFQ. ( b ) Correlation of mRNA and protein abundance changes between activated and naive T cells. ( c ) Change in protein abundance between activated and naive T cells for genes with one to four or more tandem poly(A) sites. ( d ) Correlation between the change in proximal poly(A) site use and the change in protein level. Full size image Analysis of protein expression data revealed the expected high correlation between replicate measurements ( Supplementary Fig. 4A ), and quantitative western blots confirmed the protein-level changes between naive and activated mouse T cells for ten randomly selected proteins (see Supplementary Table 6 ). Furthermore, direct comparison of mRNA levels to protein levels (iBAQ derived from LFQ) shows correlations comparable to those recently reported for a variety of tissues ( Supplementary Fig. 5C ) [40] . The changes in total mRNA levels determined as described in the previous section also correlated well with the changes in the corresponding protein levels between activated and naive T cells ( Fig. 4b ). We then asked whether genes with tandem poly(A) sites show a systematic change in protein levels compared with genes with a single poly(A) site ( Fig. 4c ) and found that for none of the groups with multiple tandem poly(A) sites could a significant difference be detected. Moreover, similar to the results obtained from the corresponding analysis on the mRNA level, we found no correlation between the change in proximal vs distal poly(A) site use and the change in protein levels ( Fig. 4d ). These data indicate that 3′ UTR shortening does not have the same consequence on the mRNA/protein abundance of all affected genes. Weak evolutionary conservation of APA To determine whether the regulation of polyadenylation at tandem poly(A) sites is evolutionarily conserved, we performed 3′ end sequencing and quantitative proteomics on naive and activated T cells obtained from a human blood donor. We found that similar to the mouse T cells, human T cells also had a pronounced increase in the use of proximal polyadenylation sites upon activation ( Supplementary Fig. 6A,B ). Also similar to the mouse T cells, the change in polyadenylation site use does not correlate with the change in gene expression, neither at the mRNA ( Fig. 5a ) nor at the protein level ( Fig. 5b ). We then investigated to what extent the changes in gene expression in the T cell activation system are conserved between mouse and human. We used the NCBI HomoloGene database [41] to infer mouse–human orthologous genes. Comparing the changes in expression of orthologous genes, we found a good correlation at both the mRNA ( Fig. 5c ) and the protein ( Supplementary Fig. 6C ) level. However, the change in the relative use of tandem poly(A) sites is not conserved. Of the 1,734 genes that show regulation by a tandem poly(A) site mechanism in both murine and human T cells, 691 genes share the same number of tandem poly(A) sites in both species. Analysis of this set of genes ( Fig. 5d ) and the bigger set of genes that generally undergo APA in both species ( Supplementary Fig. 6D ) did not reveal a correlation between the changes in the relative use of alternative poly(A) sites of orthologous genes. The set of genes that showed a strong (at least 4-fold, n =64) shift to proximal poly(A) site use in both human and murine T cells is not significantly enriched in any particular GO category. However, genes that are most enriched in this set are related to ‘stem cell division’ (adj. P =0.26) and ‘positive regulation of mitotic cell cycle’ (adj. P =0.28). Last, we investigated whether the same RBP and miRNA regulators would be affected by 3′ UTR shortening in human and mouse. We therefore predicted target sites of RBPs and miRNAs in the alternatively processed human 3′ UTRs and compared the z -scores of individual regulators between human and mouse ( Supplementary Fig. 6E,F ). Indeed, we observed some degree of conservation at this level. For example, we inferred that miRNAs of the Mir17 cluster lose more sites than expected in both systems (mouse: z -score=−2.1, human: z -score=−1.0), whereas the RBP PUM2, which has a stabilizing effect on its targets, retains more sites than expected (mouse: z -score=2.1, human: z -score=1.3). Figure 5: Evolutionary conservation of alternative polyadenylation at tandem poly(A) sites. Assessment of the impact of 3′ UTR shortening on mRNA ( a ) and protein ( b ) levels in naive and activated human T cells. ( c ) Comparison of changes in mRNA levels upon T cell activation in murine and human T cells. ( d ) Comparison of changes in poly(A) site use upon T cell activation in murine and human T cells. Only orthologous genes that showed the same number of alternative poly(A) sites in mouse and human were considered. Full size image Our analysis thus indicates that, although the process of 3′ UTR shortening in dividing cells is conserved between mouse and human, it is not highly conserved at a quantitative level and on a gene by gene basis. Furthermore, our results indicate that APA at tandem poly(A) sites contributes little to the mRNA and protein output of individual genes. Rather, what appears to be conserved is the restructuring of the RBP and miRNA interactome. That is, even though the 3′ UTR shortening of orthologous genes is poorly conserved, the RBPs and miRNAs whose targetome changes most significantly as a result of APA are the same between human and mouse. Sequencing of animal genomes revealed surprisingly small differences in gene numbers. In the years that followed, much emphasis has been placed on other factors underlying the transcriptome and proteome complexity. MiRNAs and RBPs form a vast regulatory layer whose dynamics has recently come into focus. The discovery of the systematic 3′ UTR shortening in proliferating compared with resting cells raised the question of whether this mode of RNA processing serves to bypass repression by miRNAs and generally upregulates the expression of genes with tandem poly(A) sites. Here we have combined measurements of relative polyadenylation site use with measurements of protein levels to investigate this hypothesis in the context of mouse and human T cell activation. Although we were able to demonstrate the systematic 3′ UTR shortening in both systems, we did not find a correlation between the extent of proximal polyadenylation site use and the mRNA or the protein levels. Further inferring the relative rates of decay of short and long 3′ UTR isoforms, we found that short 3′ UTR isoforms have a slightly lower decay rate compared with their long 3′ UTR isoforms. Nonetheless, the difference between isoforms appears to be small, consistent with what has been observed in mouse embryonic fibroblasts [8] and it is not systematic. Analysing the process of 3′ UTR shortening upon proliferation of mouse and human T cells, we found that although the phenomenon is conserved, there is little conservation in the set of genes that exhibit 3′ UTR shortening and in the relative change in proximal/distal processing ratios. In this respect, APA resembles alternative splicing where individual events are also poorly conserved between species such as mouse and human [42] . Two questions remain at this point unanswered. The first concerns the molecular mechanism that underlies the systematic change in polyadenylation sites upon cell proliferation. Compelling evidence has been presented that the U1 snRNP acts as a protective factor that prevents premature polyadenylation and that transient limitations in U1 snRNP abundance in specific cellular states lead to polyadenylation at proximal sites [43] , [44] . Other proteins such as the mammalian cleavage and polyadenylation factor I (CFI m ) components CFI m 25 and CFI m 68 (refs 16 , 45 ) and the poly(A)-binding protein nuclear 1 (ref. 34 ) appear to have similar effects, a reduction in their concentration leading to polyadenylation at proximal sites. In our data, the CFI m factors as well as PABPN1 appear to be downregulated at the protein level in both mouse and human T cells ( Supplementary Data 2 and 3 ). However, whether these or other factors are at work in proliferating cells remains to be determined. The second question concerns the ultimate consequence and functional relevance of the change in polyadenylation sites. Although systematic differences in the decay rates of short and long isoforms were not identified, transcript stability may still be regulated via APA, with some short isoforms having higher and others lower stability relative to their corresponding long isoforms (see for example, Gupta et al . [15] ). However, the fact that many of the proteins that lose the most or least binding sites upon APA are splicing and RNA transport factors suggests that regulatory effects may be expected at other levels. For example, one of the factors that appear to preferentially lose sites is YB-1, a marker of stress granules and processing bodies [46] . On the other hand, poly(A)-binding proteins that are involved in the nuclear export of mRNAs and many other cytoplasmic processes [47] , lose substantially fewer sites than expected. Finally, one hypothesis to consider is that 3′ UTR shortening does not have specific consequences on gene regulation. Rather, it could be a complex regulatory system, acting on long 3′ UTRs that may no longer be needed when cells are engaged in a very defined state of active proliferation. In those circumstances, the 3′ UTR shortening may act both to conserve energy, as well as to prevent the interference of complex, cell type-specific post-transcriptional regulatory networks, with the cell cycle programme. With the availability of systems that allow genetic modification of mammalian cells [48] , it may soon become possible to modify the poly(A) signals and to test the effect of expressing solely the long 3′ UTR isoforms in cells that are induced to proliferate. Isolation and activation of T cells For mouse T cells, spleen and lymph nodes were dissected from 8- to 10-week-old female C57BL/6 mice and total, untouched T cells were isolated by MACS purification (Pan T cell isolation kit from Miltenyi or the mouse T cell isolation kit from Stem Cell Technologies) according to the manufacturer’s protocol. T cells were activated for 72 h with mouse T-Activator CD3/CD28 Dynabeads (Gibco/Life Technologies) and 30 U of recombinant IL-2 (Peprotech). Corresponding unstimulated cells were from the same T cell preparations. Human T cells from single donor human blood samples were isolated with the Pan T cell isolation kit from Miltenyi and either left untreated or were stimulated with human T-Activator CD3/CD28 Dynabeads (Life Technologies) and 30 U of recombinant IL-2 from Peprotech. 3′ End sequencing and inference of poly(A) sites Murine T cell 3′ end sequencing libraries were prepared according to the original A-seq protocol [16] . To circumvent the frequently cumbersome size selection step in this protocol, we developed an improved 3′ end sequencing protocol (A-seq2) that we used for the preparation of the human 3′ end sequencing libraries (see Supplementary Methods for details). The Gene Expression Omnibus (GEO) accession number for the A-seq libraries is GSE54950. Sequencing reads were preprocessed to remove 3′ adapter sequences and mapped to the mouse genome (mm9) and human genome (hg19), respectively, with CLIPZ [21] . To ensure that only genuine 3′ ends are considered, we only used A-seq reads that contained at least four nucleotides of the adapter sequence. Based on the precise mapping of the 3′ end of reads that mapped to a unique position in the genome, we computed putative cleavage sites and their abundance at nucleotide resolution. Putative cleavage sites that had at least seven genomically encoded A nucleotides in the eight nucleotide region immediately downstream were considered likely internal priming events and were not used in further analyses. Finally, closely spaced 3′ end sites located in terminal exons of transcripts were grouped into poly(A) site clusters by applying single-linkage clustering with a distance threshold of seven nucleotides. Only those clusters that showed a minimal abundance of five A-seq reads per million were further analysed. For the mouse genome, we thereby inferred a total of 15,068 clusters with an average cluster span of 16 nucleotides. For each cluster, a representative cleavage site was chosen by ranking individual sites by their expression value in each A-seq library and then determining the overall top ranked site (majority vote over all A-seq libraries) [16] . For 3′ end sequencing of human mRNAs, we used a slightly modified A-seq procedure (A-seq2, see Supplementary Methods for details). Sequencing reads were first processed based on their expected structure from this protocol. First, only A-seq2 reads that contained three T residues at positions 5–7 (indicating the beginning of the poly(A) tail) were selected for further use. From these, randomized nucleotides at positions 1–4 at the 5′ end of the reads (needed for cluster coordination in Illumina sequencing) were trimmed together with the three Ts, thus removing seven nucleotides. The reverse complement of the remaining sequences, presumably representing mRNA 3′ ends, was then mapped to the genome. The rest of the analysis was carried out identically to the murine A-seq sequences. A total 18,918 poly(A) site clusters were inferred for the human T cell samples. Summary statistics on the number of mapped reads and tandem poly(A) sites are provided in Supplementary Tables 7 and 8 , respectively. The nucleotide profile flanking the inferred cleavage sites ( Supplementary Fig. 7A ) closely resembles the profile obtained in murine T cells ( Supplementary Fig. 2A ) and previous studies [16] . Also the distribution of polyadenylation motifs upstream of the cleavage site corresponds to the pattern observed in murine T cells ( Supplementary Fig. 7B ). In order to identify genes that show a marked change in the use of proximal and distal poly(A) sites, we first divided the region between the most proximal and most distal poly(A) site into two parts of equal length and pooled read counts of poly(A) sites in the 5′ half and in the 3′ half. For murine T cell samples, we next employed the statistical framework DEXseq version 1.8 (ref. 17 ) to identify genes that showed a change in the usage pattern between the proximal and the distal poly(A) site. A total of 157 genes were identified to undergo a significant change (adjusted P -value ≤0.05) in the use of the proximal poly(A) site. Differential gene expression and GO analysis For each gene, A-seq reads mapping to terminal exons of its associated transcript isoforms were counted. Differential gene expression analysis was performed with DESeq version 1.10 (ref. 49 ). Genes that showed a log twofold differential regulation and an adjusted P -value≤0.01 were considered as changing significantly. GO analysis of up- and downregulated genes was performed with Ontologizer version 2.0 (ref. 50 ). Prediction of miRNA and RBP target sites in murine 3′ UTRs MiRNA target predictions were obtained from the ElMMo server release 5 ( http://www.mirz.unibas.ch ). We restricted the set of target sites to conserved sites by choosing a minimal ElMMo score of 0.5. For ease of use, we mapped 3′ UTR sequences to the mouse or human genome using GMAP [51] , and converted predicted transcript coordinates of miRNA target sites to genomic coordinates. A weighted target site score was then calculated as the sum over all genes with tandem poly(A) sites, with the probability of each target site for the miRNA multiplied by the abundance of the gene’s 3′ UTR isoform in which the predicted target site was present. For each miRNA, we recorded the log 2 fold-change ( x ) of the sum of weighted target site scores in alternative 3′ UTR regions for activated over naive T cells. To assess the significance of the fold-change, we shuffled the labels of the miRNA target sites (corresponding to the cognate miRNAs) that were located in alternative 3′ UTR regions. We performed 500 randomizations and obtained the mean ( μ x ) and standard deviation ( σ x ) of the log 2 fold changes across randomized data sets. We estimated the significance of the observed log 2 fold change by the z -score defined as z =( x − μ x )/ σ x . PWMs of the binding motifs of RBPs were obtained from the CISBP-RNA database ( http://cisbp-rna.ccbr.utoronto.ca ) [32] . Only PWMs with category annotation ‘direct evidence’ in mouse or human were considered. MotEvo was used to scan murine 3′ UTRs (using a background prior of 0.99 and an UFE prior of 200) to predict evolutionarily conserved motif matches [33] . As input we provided multiple sequence alignments of nine mammalian species generated with the ElMMo pipeline [26] . Computations were performed the same way as done for miRNAs only replacing the ElMMo score with the score obtained from MotEvo. In case more than one PWM was present for a given RBP in the database, we evaluated the predicted binding sites for each of them individually, and used as background for the site randomization the sites predicted for only one representative PWM for each RBP. The representative was the PWM with the highest information content. We only report the results for PWMs that had a minimum of ten predicted sites in the alternatively processed 3′ UTR regions. Estimation of relative mRNA decay rates of short and long transcript isoforms We used the following model to estimate the relative stability of 3′ UTR isoforms. Let us assume that mRNAs are transcribed from their corresponding gene at rate c , and are processed at either the proximal or the distal poly(A) site with frequencies f and 1− f , respectively. Let μ S and μ L be the decay rates of the short and long 3′ UTR isoforms, respectively. With the dynamics of the short ( M S ) and long ( M L ) isoforms being described by the following equations d M S /d t = cf − μ S M S and d M L /d t = c (1− f )− μ L M L , and denoting by superscripts A and N the variables corresponding to activated and naive T cells, we obtain at steady state . From our 3′ end sequencing experiments, we obtain ratios of proximal-to-distal site use in the two conditions, that is, and , as well as the ratio in the overall mRNA expression between the two conditions, . With the further notation α = μ L / μ S and β = c N / c A , we can express these measured quantities in terms of the variables of the model defined above as follows . Note, that we can express the unknown frequencies of 3′ UTR processing at proximal and distal sites in the two conditions in terms of the measured ratios of proximal-to-distal site use, that is, and . Further defining x = log ( Q ), y = log ( β ), z = log ( α ) and the function , we obtain x = y + g ( R N , R A , z ) (equation 1). That is, the observed log fold-change in total mRNA levels ( x ) is a result of the log fold-change in transcription rate ( y ) and a log fold-change in the decay rate ( g ( R N , R A , z )). The latter is a function of the observed ratios of short vs long isoforms in naive and activated T cells, and of the log-ratio z of decay rates of the short and long isoforms. Note, that whereas x has been measured, the variables y and z are both unknown. Thus, we cannot uniquely determine the relative decay rates for a particular gene, without knowing the relative transcription rates for that gene in the two conditions. Reasoning that genes that are only regulated at the level of transcription and not through polyadenylation provide an upper bound on transcriptional changes, we estimate the distribution of transcription log fold-changes y from the set of genes that have only a single isoform. We found that to a good approximation, the distribution of y is a Gaussian with mean μ y =0.00154 and standard deviation σ y =0.92691, that is, . We further assume that the log-ratio of decay rates can also be approximated by a Gaussian distribution, that is, . Finally, we estimate the parameters μ z and σ z by assuming that both y and z were drawn from their respective distributions and comparing the observed mRNA fold-changes with those expected using equation 1. In particular, the log fold-changes x were measured in duplicate for each gene and this allows us to estimate the measurement error of these measurements. Let denote the pair of replicate measurements for gene i . Assuming that measurement errors are Gaussian distributed, we can estimate the variance of the measurement errors as . Given particular values of y and z , the probability to measure a given log fold-change x is given by . By multiplying this conditional probability by the prior probabilities P ( y|μ y , σ y ) and P ( z | μ z , σ z ) and integrating over both y and z we obtain the probability Note that the integral over y can easily be performed analytically to obtain This integral, however, cannot be performed analytically and we therefore carried out the integration numerically over the range μ z ±15 × σ z with MATLAB version R2012B. In order to evaluate combinations of μ z and σ z , we calculated the log likelihood of the data by a grid approach sampling values for μ z and σ z with a step size of 0.01 from −10 to 10 and 0.01 to 10, respectively. Quantitative proteomics A detailed description of the protein quantification is given in the Supplementary Methods . How to cite this article: Gruber, A. R. et al . Global 3′ UTR shortening has a limited effect on protein abundance in proliferating T cells. Nat. Commun. 5:5465 doi: 10.1038/ncomms6465 (2014). Accession codes: GSE54950 (NCBI GEO) and PXD000543 (ProteomeXchange).